Spin-torque-induced dynamics at fine-split frequencies in nano-oscillators with two stacked vortices The gyrotropic rotation around the equilibrium position constitutes the fundamental excitation of magnetic vortices in nanostructures. The frequency of this mode varies with material and sample geometry, but is independent of the vortex handedness and its core direction. Here, we demonstrate that this degeneracy is lifted in a spin-torque oscillator containing two vortices stacked on top of each other. When driven by spin-polarized currents, such devices exhibit a set of dynamic modes with discretely split frequencies, each corresponding to a specific combination of vorticities and relative core polarities. The fine splitting occurs even in the absence of external fields, demonstrating that such devices can function as zero-field, multi-channel, nano-oscillators for communication technologies. It also facilitates the detection of the relative core polarization and allows for the eight non-degenerate configurations to be distinguished electrically, which may enable the design of multi-state memory devices based on double-vortex nanopillars. Magnetic vortices in thin-film elements have been intensively studied in the past few years, as their simple structure combined with their highly non-trivial dynamic properties make them fascinating objects of research. Vortex structures benefit from a high thermal stability and develop spontaneously as flux-closure patterns. They also provide the possibility to store information by means of their two defining quantities: the sense of the circulation of the in-plane magnetization component (vorticity) and the orientation of the magnetization in the vortex core (polarity). The core region is a nanometric area where the magnetization points perpendicular to the vortex plane [1] , [2] , [3] . It results from the micromagnetic constraint to preserve the magnitude of the magnetization, irrespective of its direction. The tiny core is surprisingly important for the fundamental excitation of a vortex, the gyrotropic mode [4] , [5] , [6] , as it determines the sense of rotation. This mode is the lowest-frequency excitation known in magnetism, with frequencies far below the ferromagnetic resonance of the corresponding material. It represents the rotation of the vortex, as a whole, around its equilibrium position. The precise value of the angular frequency depends on the material and the aspect ratio of the thin-film element, and typically lies within the range of a few 100 MHz (ref. 7 ). This fundamental oscillation mode has recently been exploited in spin-torque-driven nano-oscillators (STNOs) [8] , [9] , [10] , [11] , [12] , [13] . Generally, the output frequency of STNOs can be tuned by external parameters, such as an applied field or current. These properties make STNOs particularly interesting for nanoscale communication technologies. Initial attempts of establishing tuneable STNOs used two homogeneously magnetized layers: one playing the role of a spin polarizer for the current and the other being the free, oscillating part, although these roles can hardly be separated in a very strict sense [14] , [15] , [16] . Single-domain nanopillars suffer from the disadvantage of exhibiting large linewidths (~100 MHz) due to inhomogeneous local field distributions [15] , as well as the necessity, in general, to apply external magnetic fields. STNOs exploiting the gyrotropic mode of vortices can overcome most of these difficulties, since they operate without applied field and display extremely narrow linewidths (in the order of MHz). However, their tuneability is limited, as the gyrotropic frequency is specific to the individual sample design [17] . Various groups [18] , [19] , [20] have recently reported that magnetostatic coupling induces mode splitting in vortex pairs excited by a.c. fields. Here, we demonstrate that a novel type of mode splitting arises in an STNO containing a pair of stacked vortices as polarizer–oscillator system, when using d.c. current. We find that the combined effect of spin-transfer torques, magnetostatic coupling and Oersted field introduces a fine structure, with up to eight distinct modes. Each mode belongs to a specific combination of vorticities and relative core polarities, which can be reached by applying appropriate sequences of current and field [21] . As a consequence, the system can be switched to oscillate at discrete frequencies, unlike other types of STNO devices where the frequency is tuned continuously [22] . In particular, although the discs display a coupled dynamic behaviour, our results demonstrate that one disc enslaves the other: if the current is applied such that the electrons flow from the bottom to the top disc, the sense of gyration of both vortices is solely determined by the core polarity of the top vortex. The distinctive advantage that an a priori knowledge of the mode frequencies is not required when driving the excitation with (only) d.c. currents—in contrast to the case of resonant a.c. excitation [18] , [19] , [20] —is particularly relevant for applications as high-frequency oscillators. Moreover, the fact that the output frequencies corresponding to different states are distinct can be exploited to identify the individual configurations. Consequently, this constitutes a reliable electrical read-out method for the state of the device, and thus could pave the way for designing a multi-level, non-volatile memory cell. Indeed, while spin-transfer switching has been identified as a potential write method early-on [23] , the lack of suitable methods of reading the core orientation has been the main cause hampering the development of vortex-based memory devices to-date. Sample design and static characterization We studied spin-transfer effects induced by d.c. currents in nanopillar devices with a diameter of 150 nm. The device structure included two Fe layers, with a thickness of 15 and 30 nm for the top and bottom discs, respectively, separated by a 6-nm-thin Ag spacer. The thickness difference between the two nanomagnets is important, since it lifts the degeneracy of the vortex nucleation and switching fields of the two Fe layers. Suitable sequences of current-induced Oersted fields, in combination with external magnetic fields, can therefore be designed to perform minor hysteresis loops and thus select the desired combination of vorticities. 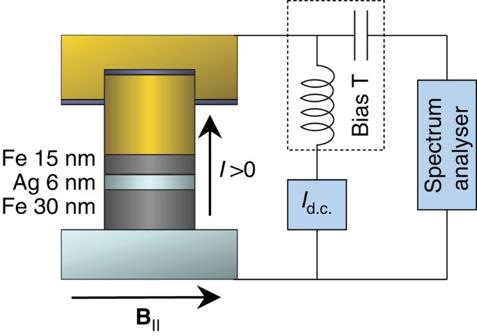Figure 1: Scheme of the experimental set-up. Schematic view of the nanopillar with layer thicknesses and the measurement set-up, including the direction of positive currentIand the in-plane component of the applied external field,B|. The d.c. sample current is provided by a constant current source, where positive current corresponds to electrons flowing from the top to the bottom electrode. High-frequency signals arising from magnetization dynamics are coupled out through a bias tee and are recorded with a spectrum analyser. Figure 1 displays a schematic representation of the experimental set-up, including the current sign convention, with positive current defined as electrons flowing from the top to the bottom layer. Figure 1: Scheme of the experimental set-up. Schematic view of the nanopillar with layer thicknesses and the measurement set-up, including the direction of positive current I and the in-plane component of the applied external field, B | . The d.c. sample current is provided by a constant current source, where positive current corresponds to electrons flowing from the top to the bottom electrode. High-frequency signals arising from magnetization dynamics are coupled out through a bias tee and are recorded with a spectrum analyser. Full size image A typical experimental magnetoresistance loop, measured with an applied current of −14 mA (corresponding to a current density of -7.9 × 10 7 A cm −2 ) is shown in Fig. 2a . Micromagnetic simulations reproduce the experimental resistance versus field scan (see Fig. 2b ), thus allowing for the magnetization states at different field values to be identified. At fields above ±300 mT, both Fe discs are saturated and their magnetic moments are parallel to each other, resulting in a low-resistance state ( Fig. 2a ). At intermediate field values, the bottom Fe layer is in a vortex state, while the top layer remains saturated. This configuration is characterized by a linear dependence of the resistance on the applied field, reflecting the continuous shift of the vortex position during the field sweep, as confirmed by micromagnetic simulations ( Fig. 2b ). The third regime is the low-resistive state observed for fields below 80 mT, where a vortex nucleates in the top disc as well, and the pillar switches into a double-vortex (DV) configuration. As the vorticities are determined by the circulation of the Oersted field, the relative orientation of the in-plane component of the magnetization in the two layers is mostly parallel. This is associated with a range of fields where the resistance level is mostly below the value corresponding to the saturated parallel single-domain configuration. The difference has been attributed to lateral electron diffusion, which occurs as the electrons propagate along the direction of the applied current [24] . In the presence of an inhomogeneous magnetization configuration, such as a vortex, this effectively causes the spin polarization of the current to decrease, yielding a lower boundary resistance at each Fe/Ag interface and thus a reduction in the resistance measured across the nanopillar. 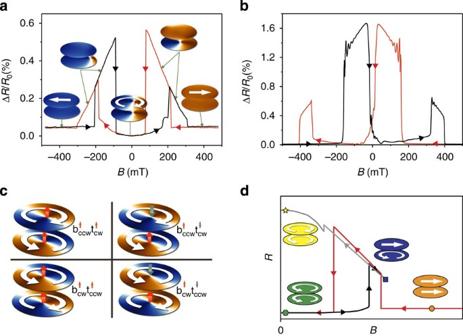Figure 2: Magnetoresistance and state preparation. (a) Change of the magnetoresistance as a function of the external magnetic field measured at a current ofI=−14 mA. As indicated by the arrows, the red curve is obtained when the field is swept from positive to negative values and the black curve for the opposite sweep direction. The magnetic field is applied in the sample plane. The insets symbolically show the magnetization states of the two ferromagnetic layers at different fields, as obtained by micromagnetic simulations. The green arrows mark in which parts of the curve the magnetization states shown by the insets occur. The white arrows display the magnetization direction, and the blue–orange colour coding represents the in-plane component of the magnetization parallel to the external field direction. (b) Dependence of the magnetoresistance change on the external field calculated from the simulations. (c) Four examples of OV–DV states with the labelling convention used in the manuscript. The labels b and t refer to the bottom and top discs, respectively. CCW and CW denote counter-clockwise and clockwise vorticity, while the red/grey arrows display the core polarities. (d) Scheme of the preparation sequence for DV states with opposite vorticities. At large external fieldBboth discs are saturated (orange dot). When reducing the field to zero in the presence of a positive current, the DV state with equal vorticities is obtained (green polygon). Then, the direction of the current is reversed. By increasing the external field to the point marked by the blue square, the vortex is expelled from the top disc. Once this configuration is obtained, decreasing the external field to zero nucleates a vortex in the top disc. This vortex has a vorticity opposite to that of the vortex in the bottom disc because the Oersted field was reversed along with the sample current. The resistanceRshows a maximum at the point marked by a yellow star. Figure 2: Magnetoresistance and state preparation. ( a ) Change of the magnetoresistance as a function of the external magnetic field measured at a current of I =−14 mA. As indicated by the arrows, the red curve is obtained when the field is swept from positive to negative values and the black curve for the opposite sweep direction. The magnetic field is applied in the sample plane. The insets symbolically show the magnetization states of the two ferromagnetic layers at different fields, as obtained by micromagnetic simulations. The green arrows mark in which parts of the curve the magnetization states shown by the insets occur. The white arrows display the magnetization direction, and the blue–orange colour coding represents the in-plane component of the magnetization parallel to the external field direction. ( b ) Dependence of the magnetoresistance change on the external field calculated from the simulations. ( c ) Four examples of OV–DV states with the labelling convention used in the manuscript. The labels b and t refer to the bottom and top discs, respectively. CCW and CW denote counter-clockwise and clockwise vorticity, while the red/grey arrows display the core polarities. ( d ) Scheme of the preparation sequence for DV states with opposite vorticities. At large external field B both discs are saturated (orange dot). When reducing the field to zero in the presence of a positive current, the DV state with equal vorticities is obtained (green polygon). Then, the direction of the current is reversed. By increasing the external field to the point marked by the blue square, the vortex is expelled from the top disc. Once this configuration is obtained, decreasing the external field to zero nucleates a vortex in the top disc. This vortex has a vorticity opposite to that of the vortex in the bottom disc because the Oersted field was reversed along with the sample current. The resistance R shows a maximum at the point marked by a yellow star. Full size image State initialization technique Depending on the magnetic history of the nanopillar, the device can support different combinations of vortex states. There are 16 possible DV configurations for the nanopillar, corresponding to all possible vorticity and core polarity combinations. The 16 DV states can be divided into states of equal and opposite vorticities (EV and OV states, respectively). For brevity, here we will focus on the OV states, although the fine structure extends to EV configurations as well ( Supplementary Figs 1 and 2 ; Supplementary Note 1 ). From the eight states in the OV configuration subset, four are displayed in Fig. 2c , which also introduces our labelling convention. As an example, b ↑ CCW t ↑ CW denotes the state where the vorticity of the bottom (b) layer is counter-clockwise (CCW), that of the top (t) vortex is clockwise (CW), and the arrows mark the orientation of their respective cores. Specific sequences of current and field applied to the nanopillar are used to initialize the desired OV–DV combination [21] . An example is depicted in Fig. 2d . Starting at positive saturation (orange dot), the field is first reduced to zero (green polygon). Here, the positive applied current induces a CCW Oersted field in the pillar and thereby selects a CCW vorticity for both layers. The applied current polarity is then reversed and the field is subsequently increased to the intermediate value denoted as the blue square, where the top Fe layer is saturated. The vortex in the bottom layer is still preserved, as this state is stable up to higher fields in this layer, due to its larger thickness. The field is then lowered again, which nucleates a CW vortex in the top disc, according to the Oersted field of the negative applied current. Correspondingly, an OV–DV configuration is obtained at the point indicated by the yellow star [25] . 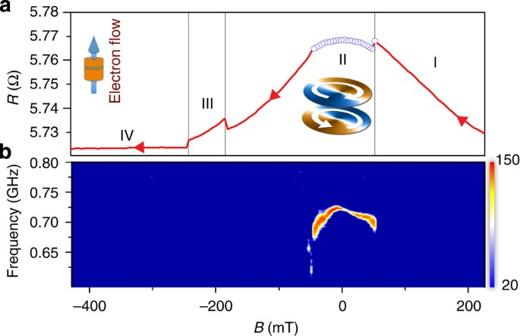Figure 3: Magnetoresistance measurement and magnetization dynamics of coupled vorticies with opposite vorticity. (a) Magnetoresistance measurement of an OV–DV state. As indicated by the red arrows along the magnetoresistance curve, the fieldBis swept from positive to negative values during the measurement of the resistanceR. At the starting point of the field sweep (region I) the magnetization in the bottom disc is in a vortex state while the top disc is still in a single-domain state. At about 50 mT, the sample switches into the OV–DV state. The inset to region II displays the vorticity combination resulting in this particular measurement. In region II, the blue circles indicate the presence of excitations simultaneously recorded during the magnetoresistance measurement, which arise from coupled gyrotropic motion of the vortices. At −180 mT, the vortex is expelled from the top disc (region III), while in region IV both discs are saturated. The inset diagram in region IV shows the direction of electron flow. (b) High-frequency spectra measured during the field sweep displayed ina. The colour code represents the power density measured in pW GHz−1in a logarithmic scale. The minimum and maximum values are shown on the colour bar. Coupled vortex dynamics induced by spin-transfer torque Figure 3 displays the simultaneously measured static ( Fig. 3a ) and dynamic ( Fig. 3b ) response of a device as a function of the applied field. At the beginning of the scan, the device is in a single-vortex state, with the top layer saturated and the bottom layer in a CCW vortex configuration, that is, the sample is in the stage of the initialization procedure referred to by the blue square in Fig. 2d . The field was swept from positive to negative values, with an applied current of −10 mA. Figure 3: Magnetoresistance measurement and magnetization dynamics of coupled vorticies with opposite vorticity. ( a ) Magnetoresistance measurement of an OV–DV state. As indicated by the red arrows along the magnetoresistance curve, the field B is swept from positive to negative values during the measurement of the resistance R . At the starting point of the field sweep (region I) the magnetization in the bottom disc is in a vortex state while the top disc is still in a single-domain state. At about 50 mT, the sample switches into the OV–DV state. The inset to region II displays the vorticity combination resulting in this particular measurement. In region II, the blue circles indicate the presence of excitations simultaneously recorded during the magnetoresistance measurement, which arise from coupled gyrotropic motion of the vortices. At −180 mT, the vortex is expelled from the top disc (region III), while in region IV both discs are saturated. The inset diagram in region IV shows the direction of electron flow. ( b ) High-frequency spectra measured during the field sweep displayed in a . The colour code represents the power density measured in pW GHz −1 in a logarithmic scale. The minimum and maximum values are shown on the colour bar. Full size image On the basis of the initial static characterization and the associated micromagnetic simulations, four distinct regions can be identified on the magnetoresistance scan, corresponding to different magnetic configurations of the device ( Fig. 3a ). The transitions between regions are marked by sharp changes in the resistance. As the field is decreased to about 50 mT, the device remains in the single-vortex state. Then, a CW vortex nucleates in the top layer (according to the Oersted field associated with the applied current). An OV–DV configuration is thus obtained. Increasing the field to negative values eventually causes the less-stable top vortex to be expelled. Finally, the vortex in the bottom layer is also ejected at about −240 mT; at higher negative fields both layers are saturated. The first high-frequency signals are resolved as the device enters the OV–DV state, with a frequency of about 700 MHz ( Fig. 3b ). The frequency increases with decreasing field, reaching a maximum of 720 MHz close to zero field. The signal then shifts to lower frequencies and finally can no longer be resolved for negative fields above −50 mT. The measured frequencies are consistent with the values expected for vortex dynamics [7] . Similar measurements were performed for various OV–DV states, each case demonstrating clear evidence of spin-torque-induced vortex dynamics, yielding a total of four modes with clearly distinct frequencies. 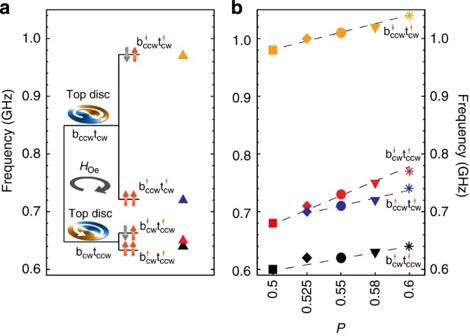Figure 4: Fine splitting of vortex gyration frequencies. (a) Experimentally obtained frequencies measured around zero field. The modes were measured at a sample current of −10 mA. The frequencies obtained by micromagnetic simulations including the spin-transfer torque are shown inbfor values of the spin-polarizationPbetween 0.5 and 0.6, where the dashed lines are guides to the eye. The simulations reveal the displayed fine structure of frequencies, which are in one-to-one correspondence with the experimentally measured values. According to the simulations, the fine structure results from two distinct splittings. The first fine splitting is defined by the relative alignment between the top vortex and the Oersted field (HOe) vorticities. This is apparent froma, where the insets indicate the vorticities of the Oersted field and the top vortex for the respective branches of the fine structure. A further hyperfine splitting is due to the relative orientation of the vortex core polarities, which are illustrated by the red and grey arrows. Note, that throughoutaandb, data points referring to identical OV–DV combinations are represented by symbols of the same colour. Figure 4a displays the fine structure of the modes measured with an applied current of −10 mA (−5.7 × 10 7 A cm −2 ) close to zero field. (The 0.64 GHz mode ( Fig. 4a ) was obtained in a more complicated way, due to a mode instability. Details are presented in Supplementary Fig. 3 and its caption.) The frequency differences between the modes are substantial, ranging from 10 to several hundred MHz. Moreover, all four modes are stable at zero applied field, implying that the mode splitting is not caused by the applied field. The fine structure is not confined to the OV states. Indeed, a similar mode splitting is also found for EV configurations (see Supplementary Figs 1 and 2 ; Supplementary Note 1 ). Figure 4: Fine splitting of vortex gyration frequencies. ( a ) Experimentally obtained frequencies measured around zero field. The modes were measured at a sample current of −10 mA. The frequencies obtained by micromagnetic simulations including the spin-transfer torque are shown in b for values of the spin-polarization P between 0.5 and 0.6, where the dashed lines are guides to the eye. The simulations reveal the displayed fine structure of frequencies, which are in one-to-one correspondence with the experimentally measured values. According to the simulations, the fine structure results from two distinct splittings. The first fine splitting is defined by the relative alignment between the top vortex and the Oersted field ( H Oe ) vorticities. This is apparent from a , where the insets indicate the vorticities of the Oersted field and the top vortex for the respective branches of the fine structure. A further hyperfine splitting is due to the relative orientation of the vortex core polarities, which are illustrated by the red and grey arrows. Note, that throughout a and b , data points referring to identical OV–DV combinations are represented by symbols of the same colour. Full size image Micromagnetic simulations To interpret the results, we performed detailed micromagnetic studies with our finite-element code TetraMag [26] . The frequencies of spin-torque-induced dynamics in a nanopillar with a similar structure and geometry to that used in the experiment were determined numerically for different combinations of vorticities and core polarities. The simulations include the local Slonczewski spin-transfer torque [27] , which depends on the current polarization P . They also account for the magnetostatic interaction between the magnetic layers and include the Oersted field contribution. Inhomogeneities of the current distribution and the resulting Oersted field have been shown to potentially influence vortex dynamics [28] . To include such effects into the simulations, we computed the current density distribution for a total current of −10 mA, considering the precise geometry of the contact leads. The result served as input for the calculation of the Oersted field used in the simulations. To obtain the mode frequency for a given OV–DV state, the spin-torque-induced dynamics was traced at each node of the finite-element mesh over a period of 100–300 ns and was subsequently Fourier transformed. The sum over all nodes provides the power spectrum of the given configuration. For each case, the lowest-frequency peak was found to correspond to the gyrotropic motion of the two vortices. Initially, numerical studies were performed for the following configurations: b ↓ CCW t ↑ CW , b ↑ CCW t ↑ CW , b ↓ CW t ↑ CCW and b ↑ CW t ↑ CCW . Additional simulations for the remaining four OV states confirmed that only the relative orientation of the vortex cores has an effect on the gyration frequency, but not their absolute direction. This is expected from symmetry considerations, since the magnetostatic coupling remains the same if both cores are simultaneously reversed. Therefore, the initial four cases yield all non-degenerate modes. Simulations were performed with different values for P , ranging from 0.5 to 0.6, since the polarization of the current is not exactly known in the experiment [24] . For most P values, spin-torque-driven dynamics is observed for all considered OV–DV states, with the exception of P =0.5, where one mode, corresponding to the b CCW t CW state with equal core polarities, is not excited for the considered system parameters and applied current. The obtained gyrotropic frequencies are shown in Fig. 4b and are found to have magnitudes similar to the measured values. As in the experiment, for each given vorticity combination, two modes are obtained—one corresponding to antiparallel core polarity and exhibiting a higher frequency and the other appearing at a lower frequency being associated with the parallel core polarity. In the experiment, the specific OV combination is set through the initialization procedure described above. However, the relative core alignment is unknown. On the basis of the simulation and considering the initialized OV combination, we attribute the b CCW t CW (b CW t CCW ) peaks measured at 0.97 and 0.72 (0.65 and 0.64) GHz to the antiparallel and parallel core alignments, respectively (Fig. 4a ). In agreement with the experimental results ( Fig. 4 ), the simulations show that the splitting between the b CCW t CW states of opposed and equal core polarities is considerably larger than in the b CW t CCW configuration. The simulations also show that generally the frequency increases with the polarization of the current, but with different slopes for the four individual modes (c.f. Fig. 4b , where the dashed lines are guides to the eye). Within each of the b CW t CCW and the b CCW t CW branches, the splitting between the two sub-branches corresponding to the two relative alignments of the cores also increases with P . Consequently, the way the frequencies of the b ↓ CW t ↑ CCW and b ↑ CCW t ↑ CW modes compare with each other depends on the exact parameters of the system considered. However, properties such as the influence of finite temperature and the spatial profile of the spin polarization are not exactly known and not included into the computation. Also, damping and saturation magnetization can have slightly different values than those considered in the simulations. This might explain why in the simulations, the frequency of the b ↓ CW t ↑ CCW state is larger than for the b ↑ CCW t ↑ CW configuration, while in the experiment the situation is reversed. Two distinct mechanisms can be identified as sources of the fine and hyperfine structure splitting, respectively. The fine splitting corresponds to the particular combination of the vorticities and their respective circulation compared with the Oersted field. Indeed, the energy of a given OV–DV state depends on three different contributions: the energy terms of the individual, non-interacting discs, the interaction between the vortices and their respective coupling to the Oersted field. Therefore, since simultaneous reversal of both vorticities leaves the first two energy contributions invariant, any associated frequency splitting must be caused by the Oersted field. The second, hyperfine splitting is connected to the relative alignment of the vortex cores. According to the simulations, for a given vorticity combination, the higher-frequency sub-branch corresponds to the antiparallel core orientation, while the lower-frequency sub-branch is associated with the case of equal polarities. Furthermore, regardless of their relative core polarities, both vortices display the same sense of gyration, which is determined by the core polarity of the vortex in the top disc. These results can be understood in the framework provided by the Thiele equation [17] , which treats the vortex core similarly to a particle in a potential. For a vortex in a single, isolated disc, the gyrational motion is described by the relation where G is the gyrovector and v is the instantaneous velocity vector of the vortex core, while W denotes the effective magnetostatic potential in which the core is moving. Accordingly, the gyration frequency f is given by where r is the trajectory radius of the circular core motion. For an isolated disc, W adopts the symmetry of the circular nanomagnet and thus exhibits a parabola-like shape with its minimum located at the disc centre. In the case of two stacked, magnetostatically coupled discs, such as considered here, the vortices mainly interact via their volume charges. These charges arise when the vortices are shifted away from the disc centres and the resulting stray field modifies the potentials W 1 and W 2 of the top and bottom discs, respectively. 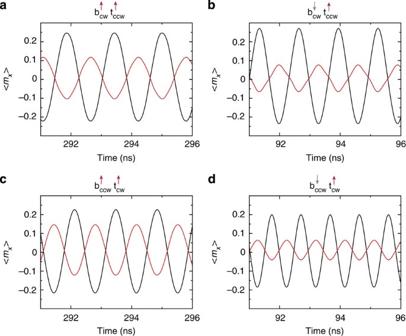Figure 5: Volume-averaged magnetization as a function of time. Time evolution of the volume-averagedx-component, ‹mx›, of the magnetization for four representative OV states (xis an axis parallel to the disc plane). These data are obtained from micromagnetic simulations. The black and the red lines refer to the magnetization in the top and in the bottom discs, respectively. (a,c) The dynamics for equally aligned vortex core polarities. (b,d) Cases of oppositely aligned cores. Compared with the states of equal core polarities, the trajectory radius of the bottom vortex is strongly reduced when the core polarities are antiparallel. Figure 5 displays the volume-averaged in-plane magnetization ( x -component) as a function of time in each disc for the simulated configurations ( P =0.6). When the cores are oriented antiparallel, the radius of the bottom vortex trajectory is always reduced compared with the corresponding configuration with parallel cores, while changes to the top vortex orbit are comparatively small, as seen comparing panels a and c with b and d in Fig. 5 . Accordingly, the stray field from the top vortex and its influence on the effective potential W 2 of the bottom vortex remain essentially the same for parallel and antiparallel cores. Symbolically, this can be denoted by , where the superscript arrows refer to the core polarities (similarly, we define ( ) as the effective potential acting on the top vortex in the case of antiparallel (parallel) core polarities). This similarity between and is also shown schematically in Fig. 6a . The reduction of the orbit radius in the case of antiparallel cores thus enables the bottom vortex to move in an energy landscape region where the potential gradient is reversed. As a result, the vortex can uphold the sense of gyration dictated by the top vortex, despite the flipped core polarity. The change in the bottom vortex trajectory radius, in turn, induces a change in the potential W 1 of the top vortex ( Fig. 6b ): such a reduction of the radius of the gyration in the bottom disc shifts the minimum of W 1 towards the disc centre, that is, the minimum of is closer to the disc centre compared with the minimum of . Thus the potential gradient at the top vortex core position is increased for antiparallel cores. This corroborates the observation that changing the relative core polarities from parallel to antiparallel leads to an increase in the gyration frequency. Figure 5: Volume-averaged magnetization as a function of time. Time evolution of the volume-averaged x -component, ‹ m x ›, of the magnetization for four representative OV states ( x is an axis parallel to the disc plane). These data are obtained from micromagnetic simulations. The black and the red lines refer to the magnetization in the top and in the bottom discs, respectively. ( a , c ) The dynamics for equally aligned vortex core polarities. ( b , d ) Cases of oppositely aligned cores. Compared with the states of equal core polarities, the trajectory radius of the bottom vortex is strongly reduced when the core polarities are antiparallel. 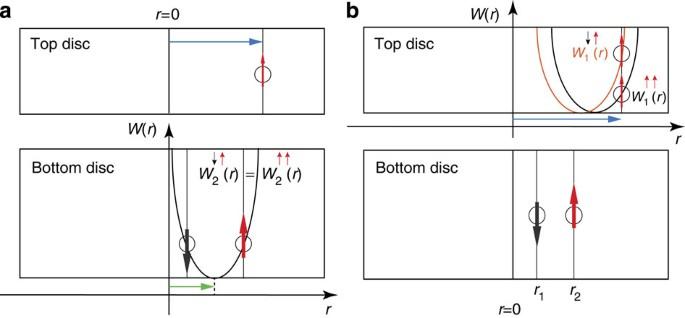Figure 6: Model for hyperfine splitting in the framework of the Thiele equation. The images show a cross-sectional side view of the two ferromagnetic discs, separated by a gap, which represents the non-magnetic spacer.r=0 defines the middle of the discs. The radius of the gyration orbitals is constant and the vortices are situated at a given distance from the disc centers, as shown by the circles. The red and grey arrows display the vortex core polarities. In the graphs,W1andW2refer to the effective magnetostatic potentials acting on the top and bottom vortices, respectively, where the arrow symbols refer to the core polarities. For example,refers to the potential acting on the bottom vortex with down polarity, when the top vortex has up polarity. (a) The simulations show that the sense of gyration of both vortices is determined by the top vortex core polarity. The lateral displacement of the top vortex along the radial directionr(displayed by the blue arrow) causes a shift of the bottom vortex-effective potential in the same direction, thus moving its minimum away from the disc centre towards the disc’s perimeter (shown by the green arrow). In the case of oppositely oriented cores, the bottom vortex reduces its orbit radius. At the reduced radius, the potential (marked by) has a negative slope, allowing the vortex to adjust its sense of gyration to that of the top vortex. (b) For a given OV combination, the different relative core polarities result in distinct gyration frequencies: parallel and antiparallel core orientations lead to different trajectory radii of the bottom vortex [(c.f. description ina)] Depending on the bottom vortex lateral position (r1orr2), the top vortex-effective potential will shift accordingly. In the case of antiparallel cores (orange curve), the potential minimum is located closer to the disc centre, resulting in a steeper potential slope at the position of the top vortex core (indicated by the blue arrow) compared with the case of parallel cores (c.f. the black potential curve). This increase in the potential slope increases the gyration frequency compared with the case of parallel cores, in agreement with the numerical results. Full size image Figure 6: Model for hyperfine splitting in the framework of the Thiele equation. The images show a cross-sectional side view of the two ferromagnetic discs, separated by a gap, which represents the non-magnetic spacer. r =0 defines the middle of the discs. The radius of the gyration orbitals is constant and the vortices are situated at a given distance from the disc centers, as shown by the circles. The red and grey arrows display the vortex core polarities. In the graphs, W 1 and W 2 refer to the effective magnetostatic potentials acting on the top and bottom vortices, respectively, where the arrow symbols refer to the core polarities. For example, refers to the potential acting on the bottom vortex with down polarity, when the top vortex has up polarity. ( a ) The simulations show that the sense of gyration of both vortices is determined by the top vortex core polarity. The lateral displacement of the top vortex along the radial direction r (displayed by the blue arrow) causes a shift of the bottom vortex-effective potential in the same direction, thus moving its minimum away from the disc centre towards the disc’s perimeter (shown by the green arrow). In the case of oppositely oriented cores, the bottom vortex reduces its orbit radius. At the reduced radius, the potential (marked by ) has a negative slope, allowing the vortex to adjust its sense of gyration to that of the top vortex. ( b ) For a given OV combination, the different relative core polarities result in distinct gyration frequencies: parallel and antiparallel core orientations lead to different trajectory radii of the bottom vortex [(c.f. description in a )] Depending on the bottom vortex lateral position ( r 1 or r 2 ), the top vortex-effective potential will shift accordingly. In the case of antiparallel cores (orange curve), the potential minimum is located closer to the disc centre, resulting in a steeper potential slope at the position of the top vortex core (indicated by the blue arrow) compared with the case of parallel cores (c.f. the black potential curve). This increase in the potential slope increases the gyration frequency compared with the case of parallel cores, in agreement with the numerical results. Full size image The above considerations explain the observed fine splitting of the modes depending on the vortex vorticities and relative core polarities. Furthermore, the analyses of both fine- and hyperfine splitting seem to assign a special role to the top vortex. The first observation concerns the Oersted field-induced frequency splitting: For a given polarity combination, the frequency is highest if the top vortex vorticity equals that of the Oersted field ( Fig. 4 ). Second, in each configuration, the top vortex dictates the sense of gyration for both vortices, that is, the dynamics of the bottom vortex is enslaved by the motion of its counterpart in the top disc. The only quantity in the system that can cause such distinguished roles of the top and bottom vortices is the direction of the electron flow. Indeed, such a symmetry breaking between the two magnetic layers is expected in view of the fundamental mechanism of spin-transfer torque: for a locally antiparallel magnetic configuration, an electron flow from the bottom to the top layer destabilizes the top layer’s magnetization, leading to excitations or switching into the parallel aligned state. The spin-torque exerted on the bottom layer, however, favours the present antiparallel configuration, that is, small deviations from the perfect antiparallel alignment with the top layer are damped away by the spin-transfer torque. Applying this picture to the OV configurations explains why the top vortex has a leading role in the coupled dynamics: In the OV configurations, the layer magnetizations are locally oriented antiparallel to each other, and the negative current used in the experiment and the simulations corresponds to electrons flowing from the bottom to the top layer, which is consistent with the above considerations. In this context it may be worth noting that while OV states are excited by negative currents, the excitation of EV states requires a positive current. In the above picture, for both cases, the top vortex is expected to take the leading role. This is also in accordance with a recent theoretical work [29] , which in either case predicts vortex gyration in the top disc. The assumption of a perfectly fixed polarizer vortex does not seem to apply in our experiment; nevertheless, the predictions in ref. 29 are consistent with the top vortex’ decisive role in the overall dynamics. In a recently reported experiment [21] on DV states of EVs, spin-torque-driven dynamics was found only in the case of opposite core polarities. This result was interpreted as evidence for the existence of a polarity-based selection rule, where the coupled vortices suppress gyration in the case of parallel cores. In contrast, our results show that spin-torque-induced vortex dynamics can occur for both relative core polarities and that the relative core orientation lifts the degeneracy of the frequency of the coupled vortex gyration. We believe that the presented fine structure property of such oscillators is attractive for applications. In particular, the property that all modes exist at zero field and can be sustained by the same current facilitates the on-chip integration. However, to exploit the effect in, for example, microwave emitters, the low output power of the present device must be increased. Higher output power could be achieved using samples based on tunnel barriers rather than metallic spacers. In this case, a suitable compromise between the desired size of the Oersted field-induced splitting and the sample diameter will need to be found, since the choice of the latter is expected to have influence on the vortex frequencies. Although probably harder to achieve, another possibility to further increase power would be a phase-locked operation of an array of such oscillators. In conclusion, we have presented a spin-torque oscillator containing two stacked magnetic vortices. We show that the variation of the gyration orbits depending on the relative core polarities in combination with the Zeeman splitting due to the Oersted field leads to a rich fine structure of oscillatory modes, most of which had remained unexplored in previous experiments. Furthermore, our experiments demonstrate the possibility to excite these modes by a d.c. driving force. The latter is an essential property for the design of spin-torque-based, integrated microwave sources as well as multi-level non-volatile memory devices. Sample preparation The sample was patterned from the multilayer stack Fe(1)/Ag(150)/Fe(30)/Ag(6)/Fe(15)/Au(50), grown on a GaAs substrate by molecular beam epitaxy (numbers in brackets refer to the layer thicknesses in nanometres). The pattering can be divided into four consecutive steps. First, the bottom electrodes are designed by optical lithography and ion beam etching. Subsequently, the nanopillar was patterned employing electron beam lithography and ion beam etching. After insulating and planarizing the nanostructures by consecutive layers of hydrogen silsesquioxane and Si 3 N 4 , a contact window was opened. Finally, the top electrode was deposited using an optical lithography step and subsequent lift-off. More details concerning the sample fabrication process are reported in ref. 30 . Measurement set-up The magnetoresistance recordings displayed in the manuscript were obtained by two-point measurements. A four-point measurement of the sample yielded about 2.35 Ω for the nanopillar at the saturated state. During the measurements of OV–DV states, the external field was tilted about 27° out-of plane to provide a bias field for the direction of the nucleating vortex cores. All fields mentioned in the text refer to the in-plane component. The bias across the sample was provided by a constant current source. D.c. and a.c. parts of the resulting signal were separated by a bias tee and recorded by a nano-voltmeter and a spectrum analyser, respectively. Figure 1 displays the measurement scheme, including the technical convention for positive current (electron flux is opposite to the arrow) as well as the definition of positive in-plane field direction used in this study. The measurements were performed at room temperature. Micromagnetic simulations The simulations are performed by numerically solving the Landau–Lifshitz–Gilbert equation with our finite-element code TetraMag [26] . The spin-transfer torque is taken into account as an additional term added to the Gilbert formulation of the equation of motion, as described in ref. 31 . The magnetization dynamics of the coupled vortex oscillators is thus described by the following explicit equation: where γ is the gyromagnetic ratio, m = M / M s is the normalized magnetization, H eff the total effective field comprising the exchange, magnetostatic, anisotropy, external and Oersted fields, α is the Gilbert damping parameter and m p is the normalized magnetization direction of the polarizer. The prefactor , where g is the Landé g-factor, μ B is the Bohr’s magneton, j the applied current density, e is the electron charge, M s is the saturation magnetization, while d refers to the thickness of the free layer. In equation (3), χ ( m · m p , P ) is a dimensionless scalar function deduced by Slonczewski [27] and depends on the angle between the magnetization of the free layer and the polarizer, and on the polarization factor P . In the experiment, both magnetic layers are subject to the spin-transfer torque. Therefore, in the simulations, the spin-transfer torque is applied to the top as well as to the bottom layer, where one layer serves as a polarizer for the other. The sign of j for the top layer is opposite to that of the bottom layer, to account for the opposed electron flow relative to the layers (in or out). The prefactor σ of the spin-transfer torque scales with the thickness of the layers. Typical material parameters of iron (Fe) are used: μ 0 M s =2.1T ( μ 0 : vacuum permeability), exchange constant A =2.1 × 10 −11 J m −1 , and K c =48 kJ m −3 (cubic magnetocrystalline anisotropy). The Gilbert damping is set to 0.02. The computational region is discretized into tetrahedra of about 2 nm edge length. The equilibrium magnetization configuration for the different OV states is simulated including the Oersted field, which is calculated considering the precise geometry of the contact leads and assuming a current of −10 mA. Simulations were performed for various values of P between 0.5 and 0.6 and for different combinations of vorticities and core polarities. The current-induced dynamics of the coupled vortex system is usually recorded for 100 ns after a dynamical equilibrium is reached. The initial oscillations are discarded from the analysis. Therefore, for some OV states the total simulation time reached as much as 300 ns. The Fourier transform of the magnetization dynamics over a period of 100 ns is calculated at each node of the finite-element mesh. The sum over all nodes provides the integral spectrum of the given configuration. A backward windowed Fourier transform is used to determine the mode profiles. We find that for each disc and for each case, the lowest-frequency peak represents the gyrotropic vortex motion, while the remaining peaks correspond to its higher harmonics. How to cite this article: Sluka, V. et al . Spin-torque-induced dynamics at fine-split frequencies in nano-oscillators with two stacked vortices. Nat. Commun. 6:6409 doi: 10.1038/ncomms7409 (2015).